Copper-catalyzed oxidative benzylic C-H cyclization via iminyl radical from intermolecular anion-radical redox relay Base-promoted C-H cleavage without transition metals opens a practical alternative for the one based on noble metals or radical initiators. The resulting carbanion can pass through radical addition to unsaturated bonds like C-N or C-C triple bonds, in which stoichiometric oxidants are needed. When in situ C-H cleavage meets catalytic carbanion-radical relay, it turns to be challenging but has not been accomplished yet. Here we report the combination of base-promoted benzylic C-H cleavage and copper-catalyzed carbanion-radical redox relay. Catalytic amount of naturally abundant and inexpensive copper salt, such as copper(II) sulfate, is used for anion-radical redox relay without any external oxidant. By avoiding using N-O/N-N homolysis or radical initiators to generate iminyl radicals, this strategy realizes modular synthesis of N-H indoles and analogs from abundant feedstocks, such as toluene and nitrile derivatives, and also enables rapid synthesis of large scale pharmaceuticals. Base-promoted C-H cleavage in the absence of transition metal catalysts, especially, without noble metals, such as rhodium, palladium, and iridium, has emerged near recently (Fig. 1a ) [1] , [2] , [3] , [4] . This approach opens a practical and cheap alternative for previously established C-H cleavage based on noble metals or radical initiators. It has been well known that carbanion can pass through radical addition to unsaturated bonds like C-N or C-C triple bonds using a metal oxidant such as Cu(II) (Fig. 1b ) [5] , [6] , [7] , [8] , [9] , [10] , [11] , [12] , [13] , [14] , [15] . Stoichiometric oxidants are needed for high turnovers [5] . The catalytic copper-mediated anion-radical relay is not possible unless an extra oxidant is presented. Thus problem emerges when in situ C-H cleavage meets carbanion-radical relay without stoichiometric high oxidation state metals or oxidants. To the best of our knowledge, the example of anion-radical oxidative relay using catalytic amount of copper salt has not been accomplished yet [5] . Fig. 1 Formation of iminyl radical from anion/radical redox relay other than N-O cleavage or initiators. a Base-promoted benzylic C-H cleavage in the absence of transition metal catalysts followed by an addition to alkenes. b Two steps/pots anion-radical relay using metal oxidants. c Methods for the generation of iminyl radicals. d This work: naturally abundant copper salt catalyzed redox C-H cyclization via iminyl radical from intermolecular anion-radical relay Full size image On the other hand, iminyl radical has been well-established as intermediates for the construction of N -containing 5- and 6-membered heterocycles including indoles and pyridines [16] , [17] , [18] , [19] , [20] , [21] . Iminyl radical is normally generated from N-O bond cleavage using either light or initiators (Fig. 1c ), which has attracted high interests of chemists with the renaissance of radical reactions in organic synthesis [17] , [22] , [23] , [24] , [25] . It has been barely reported that intermolecular carbanion-radical relay can furnish iminyl radical by catalytic transition metals. Therefore a strategy needs to be established for aforementioned challenges. As a typical 5-memebrered N -containing rings, indoles are among the most widely existing skeletons in natural products as well as in pharmaceuticals. Despite that the approaches for the synthesis indoles have been well established [26] , [27] , [28] , [29] , [30] , [31] , actually, most methods are based on the derivatives of anilines [26] , [32] , [33] , [34] , [35] , [36] , [37] , [38] , [39] , [40] , [41] , [42] , [43] , [44] , [45] , [46] , [47] , [48] , [49] , [50] , [51] , [52] , [53] , [54] , [55] , [56] , [57] , [58] , [59] , [60] , [61] , [62] , [63] , [64] , where the C-N bonds have been generally preinstalled. Therefore, we envision that a strategy through benzylic C-H addition and iminyl radical relay can enable the cyclization of toluenes and nitriles to indoles. Herein, we report our recent results (Fig. 1d ). Herein, we report our recent results in the probe of the copper-catalyzed anion-radical redox relay, we initialize the reaction by a base-promoted benzylic C-H cleavage to generate the benzyl anion A , which passes through a Cu(II)-mediated oxidation to radical B [5] . The intermolecular radical addition of B to PhCN generates iminyl radial C , which is trapped by aryl ring to form D [65] , [66] , [67] . D is reduced by Cu(I) to indoles with the regeneration of Cu(II) (Fig. 2a ). The reaction in the presence of 2 mol% CuSO 4 affords 85% of 3a (Fig. 2b ), whereas the radical trapping experiment shows that TEMPO totally inhibits the reaction with the observation of 1a -OTEMP adduct (Fig. 2c ), suggesting the radical pathway should be rational. No Ullmann-type intramolecular cyclization further proves the radical pathway (Fig. 2d ). Further investigation using palladium instead of copper salts proves no promotion effect. Therefore, CuSO 4 herein plays a crucial role of redox catalyst to generate benzylic radical from benzylic anion and enables the efficient synthesis of N-H indoles and analogs from toluene and nitrile derivatives. Fig. 2 Iminyl radical from anion-radical redox relay. a Pathway for the copper-catalyzed anion-radical redox relay. b The anion-radical redox relay of 1a and 2a in the presence of 2 mol% CuSO 4 affords 85% of 3a . c TEMPO inhibits the anion-radical redox was confirmed by the observation of 1a -OTEMP adduct. d No Ullmann-type intramolecular cyclization was observed Full size image Investigations of reaction conditions and scope The reaction conditions were optimized. 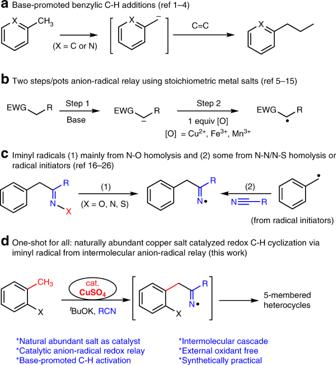Fig. 1 Formation of iminyl radical from anion/radical redox relay other than N-O cleavage or initiators.aBase-promoted benzylic C-H cleavage in the absence of transition metal catalysts followed by an addition to alkenes.bTwo steps/pots anion-radical relay using metal oxidants.cMethods for the generation of iminyl radicals.dThis work: naturally abundant copper salt catalyzed redox C-H cyclization via iminyl radical from intermolecular anion-radical relay First, various copper salts were investigated as catalysts in the cyclization of toluene 1a with nitrile 2a (Table 1 ). CuO and Cu 2 O afford similar yields (entries 2 and 3), indicating that either Cu(II) or Cu(I) might be involved in this reaction. CuSO 4 gives the best yield as 77% (entry 6). The reaction in octane is better than that in other solvents, such as dioxane, toluene, and DMF (entries 6, 9–11). Increasing the concentration results in the slight increase of yield to 81% (entries 6 and 12). Reducing the catalyst loading from 10 to 2 mol % also gives rise to the increase of yields (entries 12–13). The unreacted nitrile 2a was recovered almost quantitatively (entry 13). Palladium catalysts do not promote this reaction (entries 16–18). The reaction condition in entry 13 was chosen for the standard reaction conditions where 2 mol % of CuSO 4 was used as catalyst. Table 1 Reaction conditions Full size table With the standard reaction conditions in hand, the scope of this method was investigated. Various 2-halotoluenes were subjected to the standard conditions and the corresponding indole products were obtained (Fig. 3 ). Halogen can survive under basic conditions ( 3b , 3c , 3d , 3i , and 3l ). Such indoles are useful intermediates for further functionalization via cross coupling reactions. Starting materials with hydroxyl and carboxyl groups can directly undergo cyclization without protecting groups ( 3f and 3g ). 7-Azoindoles 3q and 3r could also be achieved by these reactions. Functional groups and protecting groups, such as halogen ( 3b-d , 3j , 3l , 3u ), (Ar)OH ( 3f ), COOH ( 3g ), MOM ( 3p ), amide ( 3l ), and ester ( 3t ), are all tolerable in this reaction. Fig. 3 Scope of methyl (het)arenes and nitriles. Reaction conditions: CuSO 4 (2 mol%), 1 (1 mmol), 2 (5 mmol), t BuOK (5 mmol), octane (0.75 mL). Extra 1 mmol t BuOK was used for 3f and 3g . a 2 (1.5 mL) was used as solvent. b Octane (3 mL). c CuSO 4 (20 mol %) was used. a 2-Iodomethyl arenes were subjected to the standard conditions. b 2-Bromomethyl arenes were subjected to the standard conditions. c 2-Chloromethyl arenes were subjected to the standard conditions Full size image Application in the synthesis of BACE1 inhibitor This indoles synthesis from nitriles and toluenes is a synthetically practical and scalable method. By this method, a BACE1 inhibitor [68] is synthesized from benzonitrile and 2-iodotoluene by our method in three steps in gram scale (Fig. 4 ). Fig. 4 Gram-scale synthesis of pharmaceuticals . a BACE1 inhibitor is synthesized from 2-iodotoluene 1a and benzonitrile 2a in gram scale using anion-radical redox relay as the key step Full size image Investigations of C3-substituted indoles and applications C3-substituted indoles can also be synthesized by this method. 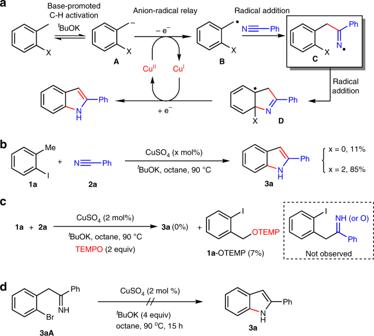Fig. 2 Iminyl radical from anion-radical redox relay.aPathway for the copper-catalyzed anion-radical redox relay.bThe anion-radical redox relay of1aand2ain the presence of 2 mol% CuSO4affords 85% of3a.cTEMPO inhibits the anion-radical redox was confirmed by the observation of1a-OTEMP adduct.dNo Ullmann-type intramolecular cyclization was observed Reaction conditions were further optimized on the basis of Table 1 (Table 2 ). Despite of the fact that even 1.5 equiv of nitrile affords 85% of 6d (entry 5), the conditions listed in entry 2 were chosen for the balance of yields and amounts of the base and nitriles. Table 2 Reaction conditions for the synthesis of 6 Full size table Indoles bearing both C3-substituents, such as phenyl, heteroaryl, phenoxyl, and phenylthio, were readily obtained (Figs. 5 , 6a–d ). These functionalized indoles are useful synthons or intermediates and are normally synthesized via C3-functionalization of indoles. For example, 2,3-diphenyl indole 6a is a key intermediate of a BACE1 inhibitor [68] . What should be mentioned is that the method for the synthesis of 3-sulfenylindoles is still limited [69] , [70] , [71] , [72] , [73] . Current method provides a powerful route to 3-sulfenylindoles ( 6d - 6p , 6s-6t ). Either aryl or alkyl substituted 3-sulfenylindoles could be achieved. C5-C7 bromo indoles are useful intermediates in organic synthesis, which were obtained in moderated to good yields ( 6m - 6o ). Plus the results in Fig. 4 , most functional groups, such as halogen, OH, COOH, amide, ester, silyl protecting group, MOM, CF 3 , nitrile, pyridine, etc, have been tolerated in this reaction. Besides 2-halogen toluenes, 2-iodo ethyl benzene is also reactive to afford the desired 3-methyl indole 6r in 55% yield. Alkyl substituted 3-sulfenylindoles are normally difficult to generate due to the instability of aliphatic nitriles under strong basic conditions. To our delight, C2-alkyl indoles could also be prepared in moderate to good yields (Fig. 6 , 6u–6z ). The yields seem dependent on the steric hindrance of nitriles ( 6u , 6v vs 6w ). Nevertheless, this reaction provides an efficient route to either aromatic or aliphatic substituted indoles. Fig. 5 Scope of C3-functionalized indoles. Reaction conditions: 5 (1 mmol), 2 (2.5 mmol), CuSO 4 (2 mol %), t BuOK (2.5 mmol), dioxane (0.75 mL). a 2 (5 mmol), t BuOK (4 mmol), octane (0.75 mL) instead of dioxane. b 2 (1.5 mL) was used as solvent. c CuSO 4 (10 mol %) was used. d Dioxane (1.5 mL). e 2 (15 mL) was used as solvent. f CuSO 4 (20 mol %) was used. g Dioxane (20 mL). h t BuOK (4 mmol). i t BuOK (4 mmol), no extra solvent. Brsm yield refers to the yield based on recovered starting material Full size image Fig. 6 Comparison between the synthesis of 3 from 1 and that from 5 . a Synthesis of 3 using a one-pot cyclization-deprotection from 5 . b Synthesis of 3 from the cyclization of 1 and 2 . c Comparison between Route 1 and Route 2 Full size image C3-phenylthio can be easily removed in the presence of 2-mercaptobenzoic acid and CF 3 CO 2 H [74] . 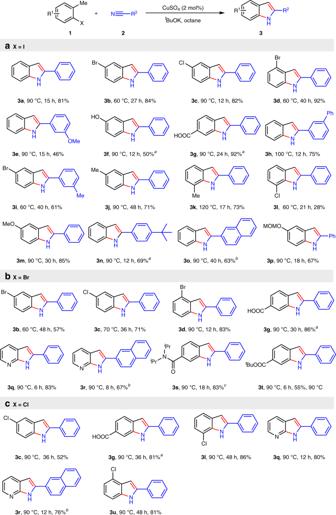Fig. 3 Scope of methyl (het)arenes and nitriles. Reaction conditions: CuSO4(2 mol%),1(1 mmol),2(5 mmol),tBuOK (5 mmol), octane (0.75 mL). Extra 1 mmoltBuOK was used for3fand3g.a2(1.5 mL) was used as solvent.bOctane (3 mL).cCuSO4(20 mol %) was used.a2-Iodomethyl arenes were subjected to the standard conditions.b2-Bromomethyl arenes were subjected to the standard conditions.c2-Chloromethyl arenes were subjected to the standard conditions Thus PhS-group can be used as a leaving group in organic synthesis. In Fig. 6 , a one-pot cyclization-deprotection synthesis of 3 either from 5 or 1 is demonstrated. Both indoles 3a and 3b were obtained in high yields via both routes, whereas indoles 3v and 3w could only be afforded by route 1 in high yields. The radical addition to nitrile is a nucleophilic process, thus the electron rich nitriles are normally less reactive. If the stability of radical intermediates are better, it gives more chance. Thio-groups are better stabilizer for adjacent carbon radicals. As a result, thio-substrate 5 is much better than 1 and some unavailable indoles from 1 and 2 can be achieved via 5 . Compound 3v is a key intermediate for a potential anti-breast cancer medicine. A potential anti-breast cancer reagent 8 is synthesized through three steps from 5f via the removal of the phenylthio in more than 10 gram-scale with overall 85% yield (Fig. 7 ) [75] . Fig. 7 Large-scale synthesis of pharmaceutical. A potential anti-breast cancer reagent 8 is synthesized from 5f in 10 gram-scale Full size image Preliminary investigations of reaction mechanism The reaction mechanism has been investigated with experimental evidence. In the reaction model in Fig. 2a , a Cu-catalyzed reaction cycle has been presented. The XPS experiments for the reaction using CuSO 4 as catalyst demonstrated both Cu(II) and Cu(I), indicating that Cu-salts have been involved in the reaction (Fig. 8 ). 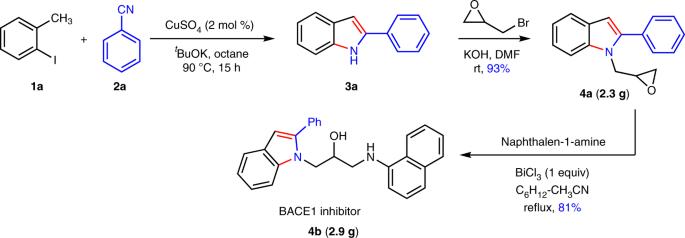Fig. 4 Gram-scale synthesis of pharmaceuticals. aBACE1 inhibitor is synthesized from 2-iodotoluene1aand benzonitrile2ain gram scale using anion-radical redox relay as the key step The iodometric determination of Cu(II) in the reaction mixture was performed using a chloro-substrate to avoid the interruption of KI generated from the reaction. By the above titration, 65% Cu(II) was determined. Therefore the reaction could possibly pass through Fig. 1a via an iminyl radical addition to aryl rings. Fig. 8 Detection of Cu(II) and Cu(I) by XPS experiments. 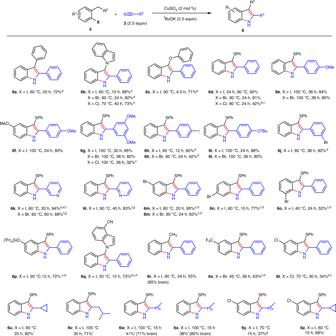Fig. 5 Scope of C3-functionalized indoles. Reaction conditions:5(1 mmol),2(2.5 mmol), CuSO4(2 mol %),tBuOK (2.5 mmol), dioxane (0.75 mL).a2(5 mmol),tBuOK (4 mmol), octane (0.75 mL) instead of dioxane.b2(1.5 mL) was used as solvent.cCuSO4(10 mol %) was used.dDioxane (1.5 mL).e2(15 mL) was used as solvent.fCuSO4(20 mol %) was used.gDioxane (20 mL).htBuOK (4 mmol).itBuOK (4 mmol), no extra solvent. Brsm yield refers to the yield based on recovered starting material a To 3a when X = I and b to 3u when X = Cl. XPS Instrument type: Thermo ESCALAB 250Xi; X-ray excitation source: monochromatic Al Ka (hv = 1486.6 eV), power 150 W, X-ray beam 500 μm; Energy analyzer fixed transmission energy: 30 eV Full size image In conclusion, we have developed a catalytic approach for the in situ generation of iminyl radicals via an intermolecular carbanion-radical redox relay using a naturally abundant copper salt as catalyst. This strategy is realized by combining a base-promoted C-H cleavage and CuSO 4 -catalyzed carbanion-radical redox relay, where CuSO 4 is a cheap and naturally abundant inorganic salt and as low as only 2 mol% catalyst loading is needed. By avoiding using N-O/N-N homolysis or radical initiators to generate iminyl radicals, this reaction provides a practical and noble metal-free access to indoles. What should be mentioned is that this method directly affords N -H indoles without any N -protecting groups, avoiding the irremovable or hard removable protecting groups in organic synthesis. This method is also a synthetically practical method, which has been readily applied in the modification of the large-scale pharmaceutical synthesis from abundant feedstocks using cheap and “green” reagents (CuSO 4 and t BuOK). General procedure The Schlenk tube charged with t BuOK (2.5–5 mmol) and CuSO 4 (0.02 mmol, 3.2 mg) was dried under high vacuum for 15 min. Octane (0.75 mL), 1 or 5 (1 mmol), and 2 (2.5–5 mmol) were added under argon and stirred at 90 °C. The resulting reaction mixture was monitored by TLC. Upon completion of the starting materials, the reaction mixture was directly purified by silica gel column to give the desired product. Procedure for XPS experiments A Schlenk tube charged with t BuOK (4 mmol, 449 mg) and CuSO 4 (0.1 mmol, 16 mg) was dried under high vacuum for 15 min. Octane (0.75 mL), 1 (1 mmol), and 2a (5 mmol) were added under argon and stirred at 90 °C for 8 h. The mixture was concentrated under vacuum and the solid was measured by XPS tests. Iodometric determination of Cu(II) in the reaction mixture A Schlenk tube charged with t BuOK (4 mmol, 449 mg) and CuSO 4 (0.1 mmol, 16 mg) was dried under high vacuum for 15 min. 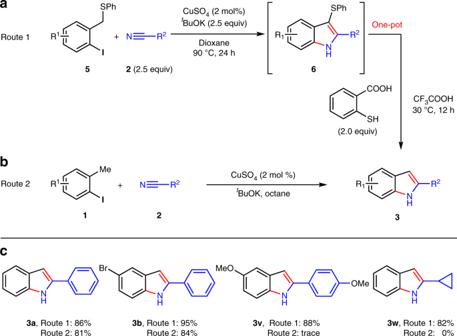Fig. 6 Comparison between the synthesis of3from1and that from5.aSynthesis of3using a one-pot cyclization-deprotection from5.bSynthesis of3from the cyclization of1and2.cComparison between Route 1 and Route 2 Octane (0.75 mL), 1u (1 mmol) and 2a (5 mmol) were added under argon and stirred at 90 °C. The reaction was stirred for 8 h and quenched by CH 2 Cl 2 and extracted with H 2 O. The aqueous phase were combined. When the pH was adjusted to 7–8, KI (8 mmol) and 5 ml of 0.5 wt% starch solution were sequentially added. 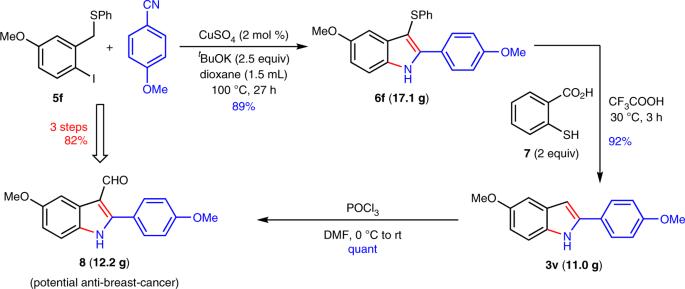Fig. 7 Large-scale synthesis of pharmaceutical. A potential anti-breast cancer reagent8is synthesized from5fin 10 gram-scale 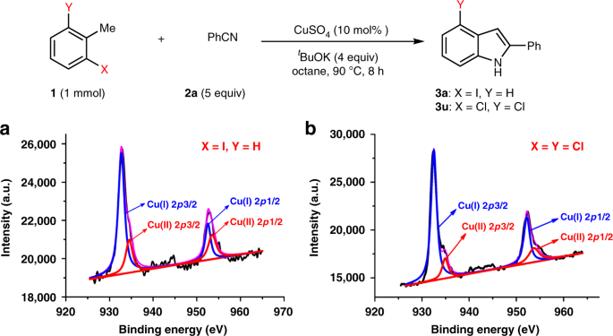Fig. 8 Detection of Cu(II) and Cu(I) by XPS experiments.aTo3awhen X = I andbto3uwhen X = Cl. XPS Instrument type: Thermo ESCALAB 250Xi; X-ray excitation source: monochromatic Al Ka (hv = 1486.6 eV), power 150 W, X-ray beam 500 μm; Energy analyzer fixed transmission energy: 30 eV Sodium thiosulfate standard titration solution [c(Na 2 S 2 O 3 ) = 0.05 mol/L] was used to titrate until the solution blue disappeared. Cu(II) was determined as 0.065 mmol (65% based on 10 mol% CuSO 4 ).